Graphene quilts for thermal management of high-power GaN transistors Self-heating is a severe problem for high-power gallium nitride (GaN) electronic and optoelectronic devices. Various thermal management solutions, for example, flip-chip bonding or composite substrates, have been attempted. However, temperature rise due to dissipated heat still limits applications of the nitride-based technology. Here we show that thermal management of GaN transistors can be substantially improved via introduction of alternative heat-escaping channels implemented with few-layer graphene—an excellent heat conductor. The graphene–graphite quilts were formed on top of AlGaN/GaN transistors on SiC substrates. Using micro-Raman spectroscopy for in situ monitoring we demonstrated that temperature of the hotspots can be lowered by ∼ 20 °C in transistors operating at ∼ 13 W mm −1 , which corresponds to an order-of-magnitude increase in the device lifetime. The simulations indicate that graphene quilts perform even better in GaN devices on sapphire substrates. The proposed local heat spreading with materials that preserve their thermal properties at nanometre scale represents a transformative change in thermal management. Self-heating is a severe problem for the high-power gallium nitride (GaN) electronic, optoelectronic and photonic devices [1] , [2] , [3] . Average temperature rise and non-uniform distribution of dissipated power in GaN transistors, leading to the formation of hotspots near device channels, result in degradation of the drain current, gain and output power, as well as an increase in the gate-leakage current and poor reliability [1] . Various thermal management solutions, for example, flip-chip bonding [4] or diamond composite substrates [5] , have been attempted. However, the hotspots, which appear due to the non-uniform dissipation of the high-power densities and relatively high thermal resistance of the substrates [6] , [7] , still limit practical applications of the nitride-based technology [1] , [2] , [3] . For example, AlGaN/GaN heterostructure field-effect transistors (HFETs) are attractive devices for high-frequency high-power communications and radar applications [1] , [2] , [8] . Owing to the large bandgap, saturation velocity of charge carriers and breakdown electrical field, AlGaN/GaN HFETs can operate at extremely high-power density of tens of W per mm of the channel width, which is unattainable with other technologies [9] , [10] . Unfortunately, at such power levels, Joule heating starts to degrade performance of GaN devices causing reliability problems. The mean-time to failure (MTTF) of GaN transistors decreases rapidly with increasing junction temperature of the devices [1] . A large number of methods have been used to improve heat removal from GaN devices. Conventional sapphire substrates with low thermal conductivity of K =30 W mK −1 at room temperature (RT) have been replaced with more expensive SiC substrates with the high thermal conductivity of K =100–350 W mK −1 at RT. However, even in GaN transistors on SiC substrate, self-heating can lead to temperature rises, Δ T , above 180 °C. The composite substrates [5] and flip-chip bonding [4] were utilized to improve the heat removal by reducing the thermal resistance on the scale of the whole wafer. Despite these efforts, the problems of the hotspots that develop near the downscaled device channels—at the nanometre and micrometre-scale—still persist. In this communication we show that the local thermal management of AlGaN/GaN HFET can be substantially improved via introduction of the additional heat-escaping channels—top-surface heat spreaders—made of few-layer graphene (FLG). The proposed heat spreaders are referred to as graphene–graphite quilts to emphasize that they patched structure and flexibility. FLG reveals an order-of-magnitude higher thermal conductivity, K =2,000 W mK −1 , than that of GaN, which ranges from ∼ 125 to ∼ 225 W mK −1 at RT [6] , [7] . The thermal conductivity of FLG is also higher than that of any metals used in the device structures. FLG films preserve their excellent phonon heat conduction properties even when they have a thickness of only a few nanometres. Contrary to FLG, the thermal conductivity of metallic thin films, which is dominated by electrons rather than phonons, degrades very fast with the decreasing film thickness. Progress in graphene-FLG synthesis and patterning on arbitrary substrates suggests that the proposed heat spreaders can become technologically and economically feasible in the near future. The demonstrated approach for the local thermal management of high-power density devices is conceptually different from conventional techniques in a sense that it specifically targets the hotspots at nanometre and micrometre scale. Instead of trying to further reduce the thermal resistance, R T , of the whole substrate, we introduce the local lateral heat spreaders on top of the GaN device structure, which provide additional heat escape channels from the hotspots. Ideally, the heat spreader should be made from material with the highest K as possible. It was recently discovered by some of us that graphene has the highest intrinsic thermal conductivity of all known materials, which increases with the lateral size [11] , [12] . From the practical applications point of view, FLG is better than single-layer graphene because its K is less subject to deterioration due to extrinsic effects, for example, defects and disorder at the interfaces [12] . In addition, FLG and thin graphite films allow for the larger in-plane heat flux through its cross-section, while still preserving graphene's mechanical flexibility. The strong anisotropy of heat conduction of FLG also means that the heat spreaders channel the heat away rather than dissipating it near the junction area. Graphene and GaN materials and devices To perform the proof-of-concept demonstration, we transferred FLG and graphite films exfoliated from the highly oriented pyrolytic graphite (HOPG) to the AlGaN/GaN devices on SiC substrate. Some of the flakes were naturally attached to thicker graphite regions. Graphite has high thermal conductivity ( K =2,000 W mK −1 ) and can be utilized both for heat spreaders and heat sinks depending on the thickness, geometry and size [12] . The fast progress in various chemical methods of large-area FLG growth [13] , [14] , [15] , [16] , stimulated by strong interest to graphene, indicates that deposition of FLG and graphite on substrates with controlled number of the atomic planes, n , will soon become a commercial technology. The latter will facilitate practical applications of FLG for heat spreading. The graphite heat sinks can also be replaced with the metallic sinks or vertical thermal vias connected to the bottom heat sink. 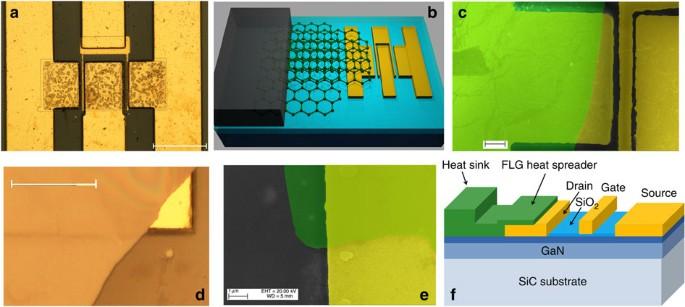Figure 1: Graphene–graphite quilts as heat spreaders for AlGaN/GaN HFETs. (a) Optical microscopy of AlGaN/GaN HFETs before fabrication of the heat spreaders. (b) Schematic of the FLG–graphite heat spreaders attached to the drain contact of the AlGaN/GaN HFET. (c) Scanning electron microscopy (SEM) image of the heat spreader transferred to the drain contact. The graphene–graphite quilt is indicated with the green colour, while metal contacts are with the yellow colour. (d) Optical microscopy image of the graphene quilt overlapping the metal drain contact and GaN surface demonstrating the heat spreader's flexibility and its close contact with the surface. (e) SEM image of the heat spreader—metal contact region and GaN surface. (f) Schematic of the device structure and the graphene–graphite quilt used in the simulation for the heat spreader optimization. Dark blue indicates the AlGaN barrier layer. Note that the FLG layer can be extended all the way to the space between the drain and the gate. The scale bars in the optical images (a) and (d) are 100 μm. The scale bars in the SEM images (c) and (e) are 10 μm and 1 μm, correspondingly. Figure 1a–f illustrates the concept of the graphene–graphite quilts as the top-surface heat spreaders and provides their microscopy images. Figure 1: Graphene–graphite quilts as heat spreaders for AlGaN/GaN HFETs. ( a ) Optical microscopy of AlGaN/GaN HFETs before fabrication of the heat spreaders. ( b ) Schematic of the FLG–graphite heat spreaders attached to the drain contact of the AlGaN/GaN HFET. ( c ) Scanning electron microscopy (SEM) image of the heat spreader transferred to the drain contact. The graphene–graphite quilt is indicated with the green colour, while metal contacts are with the yellow colour. ( d ) Optical microscopy image of the graphene quilt overlapping the metal drain contact and GaN surface demonstrating the heat spreader's flexibility and its close contact with the surface. ( e ) SEM image of the heat spreader—metal contact region and GaN surface. ( f ) Schematic of the device structure and the graphene–graphite quilt used in the simulation for the heat spreader optimization. Dark blue indicates the AlGaN barrier layer. Note that the FLG layer can be extended all the way to the space between the drain and the gate. The scale bars in the optical images ( a ) and ( d ) are 100 μm. The scale bars in the SEM images ( c ) and ( e ) are 10 μm and 1 μm, correspondingly. Full size image We used AlGaN/GaN HFETs with the layered structure consisting of 30-nm AlGaN ( ∼ 20% Al) barrier on 0.5-μm-thick GaN channel layer deposited on insulating 4H-SiC substrate. The source and drain metal contacts were made of Ti/Al/Ti/Au, while the gate electrode was made of Ni/Au. Details of the device structure and fabrication of typical AlGaN/GaN HFETs can be found in literature [8] , [9] , [10] . The gate length and widths of the devices used in this study were 3.5 and 90 μm, respectively. The large source–drain separation of 12 μm facilitated the heat spreader fabrication. The direct HOPG exfoliation on GaN/SiC substrate cannot be accomplished owing to the random nature of the process. For this reason, we applied the poly(methyl methacrylate) (PMMA)-assisted method [17] with some modifications, which allowed us an accurate placement of FLG–graphite quilts in predetermined locations on top of GaN devices. The heat spreaders were attached to the drain contacts of the devices—the closest to the hotspots—according to reported simulations [18] , [19] . We carefully avoided short-circuiting GaN devices making sure that the graphene quilts extend from the drains directly to the graphite heat sinks on the side of the devices. For the initial demonstration we used AlGaN/GaN HFETs with a large source–drain separation. At the same time, the micromanipulator, utilized for the alignment, was capable of 1–2 μm resolution sufficient for handling transistors with a smaller source–drain separation. An alignment tool with submicron resolution allows one to adapt this method for transfer graphene heat spreader to much smaller devices with submicron source–drain separation, which are typically required for high-frequency applications. The details of the FLG transfer to GaN structure are given in the Methods section. In situ temperature monitoring with Raman spectrometer The AlGaN/GaN HFETs with the heat spreaders and the reference HFETs without the heat spreaders have been wire-bonded and placed under the Raman microscope (Renishaw inVia). Raman spectroscopy was utilized both for quality control of FLG and graphite films after the transfer process and for in situ monitoring of Δ T in the powered devices. The non-contact and non-destructive micro-Raman spectroscopy technique has been previously used for T mapping in AlGaN/GaN devices by measuring the temperature-dependent shifts in the Raman peak positions [10] , [20] . We performed the measurements in the backscattering configuration under the 488-nm laser excitation. 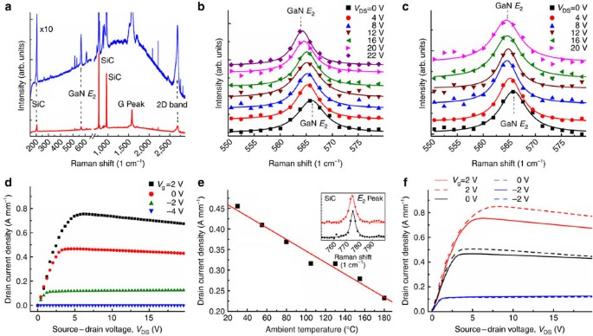Figure 2: Temperature rise in the device structure and I–V characteristics of AlGaN/GaN HFETs. (a) Raman spectrum of FLG on top of AlGaN/GaN structure on SiC substrate. The luminescence background alters the intensity ratios. To make the small peak easily distinguishable, the original spectrum (red) is shown under ×10 magnification (blue). The frequencies of SiC peaks are∼205, 610, 777 and 965 cm−1. The GaNE2peak at 567 cm−1and SiC peak at 777 cm−1are used forin situtemperature monitoring in the device channel and SiC substrate. (b) GaNE2peak shift in AlGaN/GaN HFET without the heat spreader at the power densityP=12.8 W mm−1. (c) SmallerE2peak shift in AlGaN/GaN HFET with the heat spreader indicating a reduction in the temperature rise at the same power density. (d)I–Vcharacteristics of a typical tested device without heat spreader showing self-heating effects at the high current density. (e) Saturation current in AlGaN/GaN HFET without heat spreader biased atVDS=20 V as a function of the ambient temperature. Inset shows SiCE2Raman peak used for temperature monitoring in the top portion of the SiC substrate close to the GaN channel layer. (f) Comparison ofI–Vs of AlGaN/GaN HFETs with (dashed lines) and without (solid lines) graphene–graphite quilts, indicating improvement inI–Vs in HFETs with the lateral heat spreaders. Figure 2a shows a typical spectrum from the FLG 'quilt' on AlGaN/GaN/SiC device structure. The peaks at ∼ 205, 610, 777 and 965 cm −1 are the E 2 acoustic, A 1 longitudinal acoustic, E 2 planar optical and A 1 longitudinal optical phonon modes of SiC [21] . The SiC E 2 peak at 777 cm −1 was selected for monitoring T rise in SiC substrate [22] . The measured Δ T corresponds to the top part of SiC substrate—near the GaN channel layer owing to the laser light focusing on the top surface. The temperature in the GaN channel itself was derived from the position of the narrow GaN E 2 (high) peak at 567 cm −1 . Figure 2: Temperature rise in the device structure and I–V characteristics of AlGaN/GaN HFETs. ( a ) Raman spectrum of FLG on top of AlGaN/GaN structure on SiC substrate. The luminescence background alters the intensity ratios. To make the small peak easily distinguishable, the original spectrum (red) is shown under ×10 magnification (blue). The frequencies of SiC peaks are ∼ 205, 610, 777 and 965 cm −1 . The GaN E 2 peak at 567 cm −1 and SiC peak at 777 cm −1 are used for in situ temperature monitoring in the device channel and SiC substrate. ( b ) GaN E 2 peak shift in AlGaN/GaN HFET without the heat spreader at the power density P =12.8 W mm −1 . ( c ) Smaller E 2 peak shift in AlGaN/GaN HFET with the heat spreader indicating a reduction in the temperature rise at the same power density. ( d ) I – V characteristics of a typical tested device without heat spreader showing self-heating effects at the high current density. ( e ) Saturation current in AlGaN/GaN HFET without heat spreader biased at V DS =20 V as a function of the ambient temperature. Inset shows SiC E 2 Raman peak used for temperature monitoring in the top portion of the SiC substrate close to the GaN channel layer. ( f ) Comparison of I – V s of AlGaN/GaN HFETs with (dashed lines) and without (solid lines) graphene–graphite quilts, indicating improvement in I – V s in HFETs with the lateral heat spreaders. Full size image The temperature coefficient of the SiC E 2 peak is −0.0144 cm −1 K −1 (ref. 22 ). The T dependence of the Raman peak position in GaN can be described as [23] where ω 0 is the extrapolated Raman peak position at 0 K, h is Plank's constant, k B is Boltzmann's constant, c is the speed of light, α and β are the fitting parameters [23] , [24] . The laser spot size was ∼ 1 μm. The laser power on the sample surface was well below ∼ 2 mW. As GaN and SiC are wide-bandgap semiconductors, most of the laser light (wavelength 488 nm) goes through the substrate without absorption. Our measurements indicated that taking into account the light reflection, the heating due to light absorption was on the order of ∼ 0.2 mW. Thus, the laser-induced local heating was negligible compared with the power dissipated by the transistors (above ∼ 10 W mm −1 ). The experimental data were fitted with the Lorentzian functions to determine the Raman peak positions with the spectral resolution better than 0.1 cm −1 . Figure 2b,c shows E 2 phonon peak in the Raman spectra of two AlGaN/GaN devices with and without the heat spreaders. The devices were located on the same wafer and had the same layered structure and dimensions. The laser spot was focused at the channel region between the gate and the drain, closer to the gate, where Δ T is expected to be the highest. The source–drain bias, V DS , was varied from 0 to ∼ 20 V with the 4-V intervals. The Raman peak position shifted to lower wavenumbers with increasing V DS , indicating temperature rise with increasing dissipated power owing to the Joule heating in the channel. At the power density, P , of ∼ 12.8 W mm −1 , the temperature rise, Δ T , was 92 °C for the AlGaN/GaN HFET with the graphene–graphite quilt and Δ T =118 °C in the HFETs without the heat spreader. In this specific example, the same P was achieved in the devices at 20 and 22 V due to small variations in the current–voltage characteristics ( I – V s). The corresponding Δ T measured in the top region of SiC substrate was 44 and 30 °C in the HFETs without and with the heat spreader, respectively. Our experimental data indicate that even at the moderate P , the 'graphene–graphite quilts' can help to reduce the hotspot temperature in AlGaN/GaN HFETs. Current–voltage characteristics of GaN devices Figure 2d presents I – V characteristics of representative AlGaN/GaN HFETs, while Fig. 2e shows the degradation of the saturation current with the increasing ambient temperature, T A . The tested device was completely pinched off at negative gate bias V G =−4 V. The maximum source–drain current density of I SD =0.75 A mm −1 was obtained at a positive gate bias V G =2 V. The negative-slope regions in I – V curves indicate a degradation of the carrier mobility due to Joule heating as the dissipated power increases ( Fig. 2d ). To accumulate data for Fig. 2e , the ambient temperature was changed by placing the device on a hot chuck. The saturation current density, I DS , decreases rapidly with increasing T A . For a given device I DS follows the equation I DS =0.487−0.0014× T A . The obtained I – V characteristics and the saturation current degradation with increasing T A are in agreement with literature [18] , [19] . The data illustrate the importance of temperature effects on performance of AlGaN/GaN HFETs. The inset to Fig. 2e shows Raman SiC E 2 peak for the low and high V DS in HFET without the heat spreader. Figure 2f provides direct comparison of I – V s characteristics of the HFETs with (solid lines) and without (dashed lines) graphene–graphite quilts. At V G =2 V, I SD increases from ∼ 0.75 to ∼ 0.84 A mm −1 —12% improvement—as a result of better heat removal with the top lateral heat spreaders. At V G =0 V, I SD increased from 0.47 to 0.51 A mm −1 , which is 8% improvement. At V G =−2 V, the current density remains almost the same after introduction of the heat spreader owing to the low dissipation power density at this negative gate bias. These experiments present a direct evidence of the improvement in the AlGaN/GaN HFET performance with the top-surface heat spreaders. Simulation of GaN devices with graphene quilts To rationalize the experimental results and estimate the achievable improvements in thermal management of AlGaN/GaN HFETs on different substrates, we simulated heat propagation in AlGaN/GaN layered device structures using the finite-element method (see details in the Methods and Supplementary Figs S1 and S2 ). The thickness of SiC substrate, GaN, AlGaN and SiO 2 layers were 0.4 mm, 0.5 μm, 30 nm and 10 nm, respectively. Their corresponding RT thermal conductivities were taken from literature to be 350, 160, 120 and 1.4 W mK −1 (refs 7 , 8 , 25 ). Thermal conductivity of FLG was assumed to be 2,000 W mK −1 (ref. 12 ). Thermal boundary resistance (TBR) at the GaN–substrate interface has an important role in self-heating effects [18] , [19] . The TBR value R B =1.5×10 −8 m 2 K W −1 was chosen to be consistent with the reported experimental [2] , [26] and numerical studies [27] . To make sure that the assumed K -values for the layers are reasonable, we measured the effective thermal conductivity of the whole AlGaN/GaN/SiC device structure. The measurements were performed using the 'laser-flash' technique (see Supplementary Figs S3 and S4 and the Supplementary Methods ). The effective K for the whole structure was 300±56 W mK −1 at RT. This value is in line with the data from literature for each individual layer taking into account the unavoidable contributions of TBR at several interfaces [18] . In the model, we defined the heat source at the AlGaN–GaN interface and selected the boundary conditions at the substrate bottom to be RT. To validate the developed model with the experimental data, we simulated T distribution in AlGaN/GaN HFETs without the heat spreader at P =12.8 W mm −1 . The device structure parameters corresponded to the actual tested HFET. The simulation gave Δ T =119 °C for GaN channel ( Fig. 3a ), which is in excellent agreement with the measured Δ T =118 °C. The simulated Δ T in the upper region of SiC is also in line with the experimental data. The procedure was repeated for the AlGaN/GaN HFETs with the heat spreader of the geometry similar to the experimental structure. The simulated Δ T =102 °C in GaN channel is in agreement with the measurement within the ∼ 10% uncertainty ( Fig. 3b ). An alteration of the model by adding heat dissipation through metal interconnects and probes, used in the experiments, does not significantly change the temperature distribution. The effect of the heat spreaders remains strong. 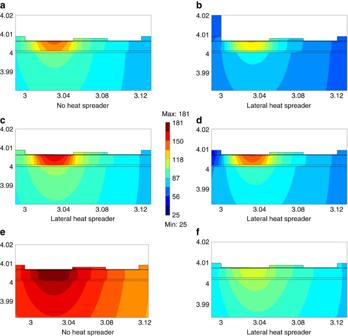Figure 3: Simulated temperature distribution in AlGaN/GaN HFETs with different graphene–graphite heat spreaders. (a) Temperature distribution in AlGaN/GaN HFET without the heat spreader showing maximumT=144 °C at the dissipated powerP=12.8 W mm−1. (b) Temperature distribution in the AlGaN/GaN HFET with the graphite heat spreader, which has sizes matching one of the experimental structures. The maximum temperature isT=127 °C at the same powerP=12.8 W mm−1. (c) Temperature profile in HFET on SiC substrate powered atP=16.8 W mm−1with the heat spreader and the heat sink located at 10-μm distance. The maximum temperature isT=164 °C. (d) Temperature profile in an identical HFET on SiC substrate powered at the sameP=16.8 W mm−1with the heat spreader and the heat sink located at 1-μm distance. The maximum temperature isT=150 °C. (e) Temperature profile in AlGaN/GaN HFET on sapphire substrate powered at 3.3 W mm−1without the heat spreader. The maximum temperature isT=181 °C. (f) Temperature profile in an identical AlGaN/GaN HFET on sapphire substrate powered at 3.3 W mm−1with the graphene–graphite heat spreader. The maximum temperature isT=113 °C. The stronger effect produced by addition of the graphene quilt is explained by the much lower thermal conductivity of sapphire. The HFET dimensions and layered structure were kept the same in all simulations. The units used in the figures are (m×10−4). The colour scheme scale is the same for all panels. The room temperature is assumed to be 25 °C. Figure 3: Simulated temperature distribution in AlGaN/GaN HFETs with different graphene–graphite heat spreaders. ( a ) Temperature distribution in AlGaN/GaN HFET without the heat spreader showing maximum T =144 °C at the dissipated power P =12.8 W mm −1 . ( b ) Temperature distribution in the AlGaN/GaN HFET with the graphite heat spreader, which has sizes matching one of the experimental structures. The maximum temperature is T =127 °C at the same power P =12.8 W mm −1 . ( c ) Temperature profile in HFET on SiC substrate powered at P =16.8 W mm −1 with the heat spreader and the heat sink located at 10-μm distance. The maximum temperature is T =164 °C. ( d ) Temperature profile in an identical HFET on SiC substrate powered at the same P =16.8 W mm −1 with the heat spreader and the heat sink located at 1-μm distance. The maximum temperature is T =150 °C. ( e ) Temperature profile in AlGaN/GaN HFET on sapphire substrate powered at 3.3 W mm −1 without the heat spreader. The maximum temperature is T =181 °C. ( f ) Temperature profile in an identical AlGaN/GaN HFET on sapphire substrate powered at 3.3 W mm −1 with the graphene–graphite heat spreader. The maximum temperature is T =113 °C. The stronger effect produced by addition of the graphene quilt is explained by the much lower thermal conductivity of sapphire. The HFET dimensions and layered structure were kept the same in all simulations. The units used in the figures are (m×10 −4 ). The colour scheme scale is the same for all panels. The room temperature is assumed to be 25 °C. Full size image Using the validated model we determined T profiles in AlGaN/GaN HFETs with different heat spreader designs ( Fig. 3c,d ). We used FLG with the number of atomic planes n =10 and the heat sink located at the distance, D , of 10 and 1 μm from the drain contact. Addition of the graphene–graphite quilt reduces temperature of the hotspot. The device structures with the closely located heat sinks offer stronger Δ T reduction ( Fig. 3d ). In the practical designs, the nearby heat sinks attached to the top-surface heat spreaders can be implemented with the vertical thermal vias. It is clear from the temperature profiles that the bulk of heat still dissipates through the substrate bottom, which serves as a global heat sink. The role of the graphene–graphite quilts is to locally redistribute the dissipated power and lower the temperature of the hotspot near the drain. The benefits of the quilts become more pronounced when one considers AlGaN/GaN HFETs on sapphire. Sapphire is a common substrate for AlGaN/GaN HFETs, which is less expensive than SiC but has lower K . Figure 3e,f shows the T profile in AlGaN/GaN HFETs on sapphire without ( Fig. 3e ) and with ( Fig. 3f ) FLG heat spreader operating at P =3.3 W mm −1 . The data show that by introducing the graphene–graphite quilt with the heat sink at D =10 μm one can achieve a drastic 68 °C reduction in the hotspot temperature. The experimentally observed and computationally predicted reduction in Δ T can lead to more than an order-of-magnitude increase in MTTF of GaN HFETs [1] . To elucidate the scientific and technological importance of our findings it is illustrating to compare the thermal properties of FLG with those of metals, which can also be used as heat spreaders. It is well known that the thermal conductivity of metal films rapidly decreases with the film thickness [28] , [29] , [30] , [31] . For many technologically important metals, for example, aluminium, copper or gold, the thermal conductivity of the metal film, K F , constitutes only ∼ 20% of the thermal conductivity of bulk metal, K M , at the film thickness H ≈100 nm. For example, the thermal conductivity of the gold film on etched Si for H approaching the electron mean free path Λ≈41 nm is K F ≈0.2× K B (ref. 30 ). The expected down-scaling for aluminium films would give K F =26–48 W mK −1 considering that the bulk RT K M value for aluminium ranges from ∼ 130 to 240 W mK −1 , depending on its purity and quality. The drastic degradation of the heat conduction properties of metal films is due to the increased electron scattering from the rough surfaces of the films and the polycrystalline grain boundaries. The surface roughness of thin metal films is usually rather high [29] leading to stronger diffusive phonon scattering from interfaces. From the other side, despite being highly electrically conductive, graphene and graphite reveals thermal conduction, which is dominated by the acoustic phonons owing to the strong sp 2 bonding of their crystal lattices [11] . It has been shown both experimentally and theoretically that the thermal conductivity of FLG is close to the bulk graphite limit of ∼ 2,000 W mK −1 all the way to the few-nanometre thickness. The intrinsic thermal conductivity of FLG can increase even further when the number of atomic planes is below n =4 (ref. 12 ). In the case of the extrinsically limited thermal transport, for example, via phonon—boundary or phonon—defect scattering, the thermal conductivity of FLG is still close to that of bulk graphite. Detailed experimental studies found that even when FLG is embedded between two SiO 2 amorphous layers with rough interfaces the bulk graphite's thermal conductivity limit is recovered at the FLG thickness of only 10 nm in spite of the presence of disorder [32] . For this reason, the thermal conductivity of FLG is larger than that of thin metal films almost by two orders of magnitude leading to substantial differences in the heat fluxes when these materials are used as heat spreaders. The benefits of FLG as the material for heat spreaders can become even more pronounced if one uses isotopically pure graphene grown by the chemical vapour deposition (CVD). It has been recently reported that the thermal conductivity of the isotopically engineered graphene is a factor of two higher than that of the natural graphene, which translates to an increase by ∼ 1,000 W mK −1 near RT [33] . The anisotropic nature of thermal conductivity in FLG is also a positive characteristic, which allows one to channel the heat away from the heat-sensitive areas other than dissipating it in their vicinity. To test the differences between FLG and metal directly we simulated temperature distribution in AlGaN/GaN HFET structure with the metal heat spreaders using our experimentally validated numerical model. Considering the best case scenario for the metal, we assumed its thermal conductivity to be 320 W mK −1 , which corresponds to a thick gold or copper film. The layered structure and geometry was selected to be exactly the same as in the HFETs with graphene heat spreaders. It was found that in AlGaN/GaN HFET with the metal heat spreader, the device temperature increased by ∼ 10 °C as compared with the case with the FLG heat spreader. This change is significant considering that the hotspot temperature reduction by ∼ 20 °C corresponds to an order of magnitude increase in MTTF of GaN HFETs. Using more realistic values for thermal conductivity of thin metal films would make the difference in thermal management performance between FLG and metals even stronger. The cost of sp 2 carbon unlike that of copper or other technologically important metals is expected to lower as the technology matures. Our experimental data indicate that thermal coupling between FLG fabricated on top of AlGaN/GaN HFET device structure is sufficient for heat transfer from the hotspot inside the device to the top FLG heat spreader. It is reasonable to assume that FLG grown directly on the layered structure will be coupled stronger thermally. One should be mentioned here that it was previously found that the Kapitza TBR between graphene or graphite and various substrates is relatively small, on the order of ∼ 10 −8 Km 2 W −1 at RT and does not strongly depend on the interfacing material [34] , [35] , [36] . Another observation from our experimental studies is that the thermal conductivity of FLG remains high after processing, micromanipulations, transfer to another substrate and coupling to metal electrodes. We finally note that practical applications of graphene quilts can be implemented with FLG grown and patterned directly on the GaN or other substrates rather than with FLG transferred to GaN device structures. Fast progress in graphene growth by CVD and other techniques [15] , [37] , [38] , [39] , its patterning and quality control [40] make this prospect feasible. The exotic electrical and thermal properties of graphene stimulated interest to CVD growth of FLG on various substrates, which, in turn, can make integration of FLG–graphite with various semiconductors and metals a reality in a short time. The proposed FLG heat spreaders can become important industry-scale thermal application for graphene and related sp 2 carbon materials [41] . They can also provide an additional impetus for further development of the nitride-based technology. Similarly with graphene–FLG applications as fillers in the thermal interface materials [42] , [43] , the FLG quality for heat spreaders does not need to be as high as that for the electronic applications. Recent demonstration of direct low-temperature growth of synthetic diamond on GaN [44] can lead to the development of heterogeneous FLG-diamond lateral heat spreaders, where the diamond layers provide electrical insulation and additional heat spreading [45] . The described thermal management of the hotspots at the micro- and nanometre length scale versus packaging level thermal solutions represents a transformative change, which can only be possible with the materials that preserve their excellent heat conduction properties even when they are structured at the nanometre scale. FLG transfer to GaN/SiC substrate It was required to transfer FLG films on top of AlGaN/GaN devices placing them precisely at the drain electrode location. The channel region between the gate and the drain generates most of heat. The FLG film should not touch other exposed electrodes and should be connected to larger graphite bars acting as the heat sinks. We adopted a method, which utilizes PMMA as the supporting membrane for transfer to the desired location [17] , but modified it for our purposes ( Fig. 4 ). The innovation to the transfer procedure, which we introduced, is that we coat the substrate with PMMA before exfoliation of graphene on top of it. As a result, only one side of FLG contacts another material reducing possible residue. 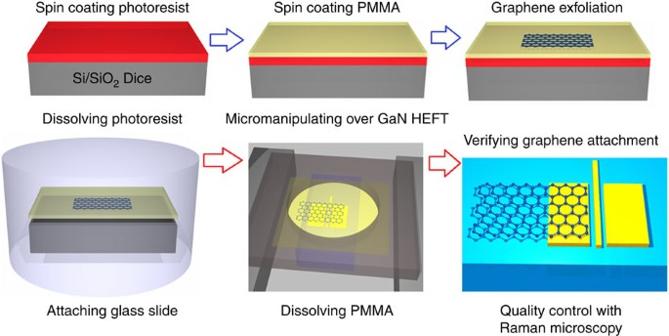Figure 4: Transfer of FLG films to exact locations on AlGaA/GaN HFET device structure. The first set of steps, indicated by blue arrows, includes spin coating of the photoresist and PMMA, followed by FLG exfoliation on top of PMMA. The second set of steps, indicated by red arrows, consists of dissolving photoresist and attaching graphene to glass slides. The slide is micromanipulated over AlGaN/GaN HFET to exact location under optical microscope. Dissolution of PMMA leaves FLG film in the desired location. Micro-Raman inspection confirms the number of layers and the quality of FLG after the transfer process. Figure 4: Transfer of FLG films to exact locations on AlGaA/GaN HFET device structure. The first set of steps, indicated by blue arrows, includes spin coating of the photoresist and PMMA, followed by FLG exfoliation on top of PMMA. The second set of steps, indicated by red arrows, consists of dissolving photoresist and attaching graphene to glass slides. The slide is micromanipulated over AlGaN/GaN HFET to exact location under optical microscope. Dissolution of PMMA leaves FLG film in the desired location. Micro-Raman inspection confirms the number of layers and the quality of FLG after the transfer process. Full size image First, we spin coated a layer of photoresist (Shipley 1813) with 3,500 r.p.m. and baked it at 110 °C for 90 s. The substrate was then exposed with ultraviolet light. A second layer of polymer PMMA was spin coated with 3,500 r.p.m. and baked at 130 °C for 90 s. We followed with the mechanical exfoliation from HOPG to produce graphene on the substrate. After the coating procedure, FLG films (even the single-layer graphene) can be optically identified under the microscope. Completing the procedure, we immersed the samples in photoresist developer (AZ400/H 2 O=1:4) and dissolved the photoresist. The PMMA membranes were floated in the liquid. We used metal slides with the holes to attach the PMMA membranes. Note that the locations of the FLG films were roughly estimated to make sure that they fell into the holes. After removing the membranes from the liquid, the metal slides were mounted on a micromanipulator, which was used for alignment. We were able to see the FLG films through the hole under the optical microscope and adjust the position of the substrate to place graphene on top of the desired location. The PMMA membranes were dissolved by hot acetone leaving FLG films attached to the substrate. Simulation of heat dissipation in the device structure A finite-element method has been used to study heat diffusion in the investigated AlGaN/GaN HFET structures with and without the graphene heat spreaders. The schematic of simulated device structure is shown in Fig. 3 . The overall dimension of the simulation domain was 600 μm, which is much larger than the device feature size. The thickness of SiC, GaN, AlGaN and SiO 2 layers were 400 μm, 500 nm, 30 nm and 10 nm, respectively. Their corresponding thermal conductivities were taken from literature to be K =350, 160, 120 and 1.4 W mK −1 , respectively. The thermal resistance of the resulting structure with assumed K values was in agreement with the measurements of the effective thermal conductivity of the device structure. The thickness of the gate electrode was 120 nm and the thickness of the drain and source electrode was 240 nm. Considering that the main component of the electrodes was gold, we used K =320 W mK −1 at RT. The heat source had rectangular shape with the 4-μm width and 10-nm thickness. It was placed at the interface of AlGaN and GaN layers, at the drain-gate opening, near the gate side. TBR at GaN–substrate interface affects self-heating effect in GaN transistors. TBR was modelled with a virtual thermal isolation layer of the small thickness, h , between the GaN channel and SiC substrate. The effective thermal conductivity of this layer was defined as K=h/R B , where R B is TBR at the GaN–SiC interface. We adopted R B =1.5×10 −8 m 2 K W −1 from the reported experimental studies [24] , [25] , [26] . The heat diffusion was simulated by numerically solving the Fourier's equation with proper boundary conditions. The bottom of SiC substrate and the left side of graphene heat spreader were kept at a constant temperature T 0 =25°C. The external surfaces were modelled as insulated from the environment. The triangular mesh was generated through the investigated structure for the numerical solution ( Supplementary Fig. S1 ). After validating this model with the experimental data we simulated temperature profiles in AlGaN/GaN HFETs with and without graphene–graphite heat spreaders. The simulation results were in agreement with the experimental data within the 10% uncertainty. To estimate the optimized conditions that could be achieved with the graphene–graphite quilts, we carried out several simulations with different heat spreader designs. In most of the simulation runs we assumed FLG films consisting of ten layers of carbon atoms. The location of the top surface heat sink was at the distance D selected in the range from 1 to 50 μm. The dependence of Δ T with the distance to heat sink is shown in the Supplementary Fig. S2 . The device structures with the closely located heat sinks offer stronger Δ T reduction. At D =1 μm, the maximum Δ T= 32 °C decrease can be obtained for a given power density and device structure. In the practical designs, the nearby heat sinks attached to the top-surface heat spreaders can be implemented with the vertical thermal vias. How to cite this article: Yan, Z. et al . Graphene quilts for thermal management of high-power GaN transistors. Nat. Commun. 3:827 doi: 10.1038/ncomms1828 (2012).